Hace1 controls ROS generation of vertebrate Rac1-dependent NADPH oxidase complexes The Hace1-HECT E3 ligase is a tumor suppressor that ubiquitylates the activated GTP-bound form of the Rho family GTPase Rac1, leading to Rac1 proteasomal degradation. Here we show that, in vertebrates, Hace1 targets Rac1 for degradation when Rac1 is localized to the nicotinamide adenine dinucleotide phosphate (NADPH) oxidase holoenzyme. This event blocks de novo reactive oxygen species generation by Rac1-dependent NADPH oxidases, and thereby confers cellular protection from reactive oxygen species-induced DNA damage and cyclin D1-driven hyper-proliferation. Genetic inactivation of Hace1 in mice or zebrafish, as well as Hace1 loss in human tumor cell lines or primary murine or human tumors, leads to chronic NADPH oxidase-dependent reactive oxygen species elevation, DNA damage responses and enhanced cyclin D1 expression. Our data reveal a conserved ubiquitin-dependent molecular mechanism that controls the activity of Rac1-dependent NADPH oxidase complexes, and thus constitutes the first known example of a tumor suppressor protein that directly regulates reactive oxygen species production in vertebrates. HACE1 (HECT domain and Ankyrin repeat Containing E3 ubiquitin-protein ligase 1), a tumor suppressor gene originally cloned from inactivating chromosome 6q21 breakpoints in human Wilms’ tumor, is found exclusively in vertebrates and is widely expressed in human tissues [1] . It is epigenetically inactivated in human Wilms’ tumors and several other tumor types [1] , [2] , [3] , [4] , [5] , [6] . In a recent study, loss of Hace1 expression is associated with neuroblastoma progression and predicts poor overall patient survival [2] . These observations are consistent with HACE1 functioning as a chromosome 6q21 tumor suppressor gene. Indeed, Hace1−/− mice develop late-onset (18–24 months) spontaneous tumors across all three germ layers [6] . Tumor development is dramatically accelerated by DNA damage inducing agents such as low-dose ionizing radiation (IR) or the DNA alkylating agent, urethane [6] , but the basis for this hypersensitivity is not understood. Hace1 reduces in vitro and in vivo cell cycle progression of diverse tumor cell lines such as KRAS-transformed NIH3T3 fibroblasts or human Ewing sarcoma SKNEP1 cells [6] . Re-expression of Hace1 in these cells blocks in vitro and in vivo proliferation, particularly after cell stress such as IR, nutrient deprivation or contact inhibition. This correlates with marked repression of cyclin D1 protein levels [6] , a key G1-S progression factor [7] . After serum deprivation or IR, Hace1 blocks cell cycle re-entry in an E3 ligase-dependent manner through failure of cells to re-express cyclin D1, while other cyclins are unaffected. This occurs in a ligase-dependent manner, although Hace1 does not itself target cyclin D1 for ubiquitylation [6] . D-type cyclins have well-established roles in oncogenesis, and overexpression of cyclin D1 is reported in diverse human malignancies [8] . Knockdown of endogenous Hace1 in HEK293 cells (which express high endogenous Hace1 levels) by RNA interference stabilizes cyclin D1 protein levels, and ectopic expression of Hace1 blocks cyclin D1 expression, as well as in vitro and in vivo cell cycle progression of Hace1-deficient human tumor cell lines [6] . Currently, the only known Hace1 E3 ligase substrate is the GTP-bound form of the Rho GTPase, Rac1. The latter is bound and ubiquitylated by Hace1 at lysine-147 (Lys-147), leading to Rac1 proteasomal degradation and reduced cell motility in response to cytotoxic necrotizing factor-1 (CNF1) or hepatocyte growth factor [9] , [10] . Rac1 localizes to various cellular compartments and regulates multiple processes including cell motility [11] , protein translation [12] , stress signaling [13] , proliferation [14] and reactive oxygen species (ROS) generation [15] , [16] . How Rac1 activity orchestrates such diverse functions is poorly understood, but evidence suggests that subcellular localization of activated Rac1 is a critical factor [15] , [17] , [18] . Hace1 co-localizes with a small fraction of total Rac1 in cells, corresponding to the active (GTP-bound) form of the protein, at any given time [9] . Moreover, a second class of E3 ligases, X-linked and cellular inhibitors of apoptosis IAP1 (XIAP and c-IAP1, respectively) directly bind Rac1 in a nucleotide-independent manner and promote Lys-147 polyubiquitylation and proteasomal degradation [19] . This suggests that different E3 ligases might target Rac1 at distinct subcellular sites. In the current study, we sought to uncover why Hace1 deficiency confers in vivo hypersensitivity to IR and urethane, and whether this is linked to Rac1 targeting by Hace1. Besides the mitochondria, the main sources of cellular ROS are plasma membrane and endosomal nicotinamide adenine dinucleotide phosphate (NADPH) oxidase complexes [20] . These are the only known mammalian enzymes exclusively dedicated to the production of superoxide, which is rapidly converted to H 2 O 2 in the cell [21] . The NADPH oxidase holoenzyme consists of transmembrane catalytic cell type specific Nox subunits 1–5 (predominantly Nox1 and Nox2 in epithelial and mesenchymal cells), the transmembrane p22phox protein, and the cofactors p47phox, p67phox, NOXA1 and NOXO1 (ref. 21 ). Rac1 GTPase binds NOXA1 within the complex and this is required for activation of Nox1, 2 and 3-containing NADPH oxidase enzymes [16] , [21] . Accordingly, we hypothesized that increased ROS in Hace1-deficient cells might derive from hyperactivation of NADPH oxidase due to Rac1 stabilization. Here we show that Hace1 binds and ubiquitylates Rac1 when the latter is associated with NOXA1 at the NADPH oxidase complex, thus blocking ROS generation by the complex. Moreover, loss of Hace1 in human tumors and cell lines, mice and zebrafish results in ROS-induced DNA damage and cyclin D1 induction, each of which depends on Rac1 and NADPH oxidase activity. Taken together, our results reveal Hace1 as the first known negative regulator of NADPH oxidase, and highlight the role of deregulated NADPH oxidase activity in ROS-induced DNA damage and cell cycle progression. Hace1 deficiency leads to chronic oxidative stress IR and urethane, which both dramatically accelerate tumor formation in Hace1 −/− mice [6] , are each known to induce high levels of ROS, particularly H 2 O 2 (refs 22 , 23 ). We therefore speculated that Hace1 might itself regulate cellular ROS levels. Indeed, measurement of ROS levels in control and Hace1 −/− MEFs with 2′,7′ dichlorodihydrofluorescein diacetate (DCFDA) [24] showed a marked baseline elevation of ROS in Hace1 −/− MEFs, which could be almost completely reversed by re-expression of wild-type ( wt) Hace1 ( Fig. 1a ). Increased ROS was also detected in Hace1 −/− MEFs with a second sensor, dihydroethidium (DHE), which is converted to the red fluorescent compound oxyethidium in vitro and in vivo in the presence of ROS [25] ( Fig. 1b and Supplementary Fig. S1a ). Staining with MitoSoxRed, which specifically measures mitochondrial ROS, was largely unchanged between Hace1 +/+ and Hace1 − / − cells. We then used nitrotetrazolium blue (NTB) to visualize ROS in Hace1−/− and +/+ MEFs, which clearly demonstrated formazan dots along the cell membranes and also in punctate dots within the cytoplasm in Hace1−/− cells ( Supplementary Fig. S1b ). These data are consistent with Hace1 deficiency resulting in massive accumulation of ROS from membrane-associated NADPH oxidase complexes, but it is possible that under chronic ROS accumulation additional ROS sources are activated, such as mitochondria. To confirm a role for Hace1 in regulating ROS levels, we knocked down Hace1 expression in human embryonic kidney (HEK) 293 cells using two non-overlapping short interfering RNAs (siRNAs) ( Supplementary Fig. S1c ). Total ROS levels increased by 4- to 6-fold in Hace1 knockdown (kd) cells compared with controls ( Fig. 1d ). Moreover, all organs isolated from Hace1 −/− mice showed dramatic increases in ROS compared with those of littermate controls ( Fig. 1e ). Therefore, Hace1 deficiency in mammalian cells leads to chronic high ROS levels in vitro and in vivo . To determine whether Hace1 regulation of cellular ROS is conserved, we identified the hace1 homologue in zebrafish, which displays 74.7% DNA sequence homology and 88.9% protein identity with human HACE1 ( Supplementary Fig. S2a,b ). A hace1 morpholino was designed to knock down hace1 expression ( Supplementary Fig. S2c,d ), and zebrafish embryos were incubated over 1–7 days with the H 2 O 2 -specific probe, pentafluorobenzenesulphonyl fluorescein, which is converted to a fluorescent form by H 2 O 2 (ref. 26 ). A significant increase in ROS levels was observed in hace1 morpholinos compared with control morpholinos or uninjected embryos ( Fig. 1f ). This could be completely rescued by addition of the broad flavoenzyme inhibitor diphenylene iodonium (DPI) [27] ( Fig. 1f ) or the panoxidase inhibitor, apocynin (APO) [28] ( Supplementary Fig. S2e ), both of which have well-documented antioxidant activities. Together, these data demonstrate that Hace1 deficiency results in massive accumulation of ROS in vertebrates. 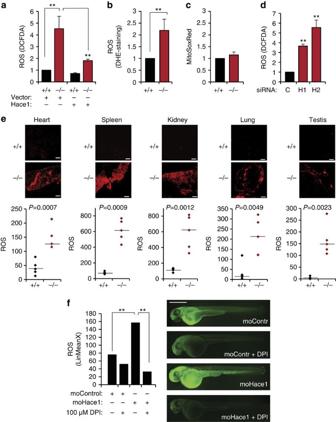Figure 1: Hace1 deficiency leads to elevated levels of ROS. (a) MEFs derived from wild-type (+/+) or Hace1 knockout (−/−) mice were transfected with the HA-vector (V) or HA-Hace1 (H) 48 h and analyzed for ROS content by the DCFDA assay. (b) MEFs analogous toawere incubated with 10 μM DHE for 30 min, analyzed for oxyethidium staining by a 595-nm enabled fluorescence microscope and quantified using ImageJ algorithm. (c) MEFs as inawere analyzed for mitochondrial derived ROS by the MitoSoxRed probe (Invitrogen). (d) HEK293 cells were transfected with control siRNA (C) or two siRNAs targeting Hace1 (H1 and H2) for 72 h and analyzed as inb. (e) Snap-frozen samples of the indicated tissues specimens from Hace1 wild-type (+/+) and knockout (−/−) mice were cut in 20 μm sections using a cryostat at −20 °C, incubated with 10 μM DHE for 30 min and analyzed as inb. The p values were generated using student’s two-tailedt-test for equal variance. Scale bars, 20 μm. Horizontal lines in the graphs represent median values of quantification by ImageJ algorithm. (f) Representative images of 48 h post fertilization (hpf) casper zebrafish control (mC) and hace1 (mH) morphants stained for ROS using pentafluorobenzenesulphonyl fluorescein. Both control and Hace1 morphants were left untreated or incubated with DPI as indicated, before being analyzed for ROS-induced fluorescence by FACS. For all panels when indicated, **P<0.01 (Student’s two-tailedt-test for equal variance); Error bars represent s.e.m. of at least three independent experiments. Scale bar, 0.5 mm. Figure 1: Hace1 deficiency leads to elevated levels of ROS. ( a ) MEFs derived from wild-type (+/+) or Hace1 knockout (−/−) mice were transfected with the HA-vector (V) or HA-Hace1 (H) 48 h and analyzed for ROS content by the DCFDA assay. ( b ) MEFs analogous to a were incubated with 10 μM DHE for 30 min, analyzed for oxyethidium staining by a 595-nm enabled fluorescence microscope and quantified using ImageJ algorithm. ( c ) MEFs as in a were analyzed for mitochondrial derived ROS by the MitoSoxRed probe (Invitrogen). ( d ) HEK293 cells were transfected with control siRNA (C) or two siRNAs targeting Hace1 (H1 and H2) for 72 h and analyzed as in b . ( e ) Snap-frozen samples of the indicated tissues specimens from Hace1 wild-type (+/+) and knockout (−/−) mice were cut in 20 μm sections using a cryostat at −20 °C, incubated with 10 μM DHE for 30 min and analyzed as in b . The p values were generated using student’s two-tailed t -test for equal variance. Scale bars, 20 μm. Horizontal lines in the graphs represent median values of quantification by ImageJ algorithm. ( f ) Representative images of 48 h post fertilization (hpf) casper zebrafish control ( mC ) and hace1 ( mH ) morphants stained for ROS using pentafluorobenzenesulphonyl fluorescein. Both control and Hace1 morphants were left untreated or incubated with DPI as indicated, before being analyzed for ROS-induced fluorescence by FACS. For all panels when indicated, ** P <0.01 (Student’s two-tailed t -test for equal variance); Error bars represent s.e.m. of at least three independent experiments. Scale bar, 0.5 mm. Full size image Rac1 is required for ROS induction in Hace1-deficient cells As increased ROS in Hace1-deficient cells is not mitochondrially derived, we speculated that Hace1 might regulate NADPH oxidase complexes, another major source of cellular ROS. First, we analyzed ROS levels in Hace1 −/− MEFs after treatment with 2-Acethylphenothiazine (ML171), which specifically inhibits Nox1-containing NADPH oxidases [29] , and two agents that block cellular ROS accumulation, DPI [27] and APO [28] . All three inhibitors reduced ROS levels as effectively as wt Hace1 re-expression ( Fig. 2a and Supplementary Fig. S3a ). We then analyzed whether genetic loss of NADPH oxidase components influences ROS levels in Hace1-deficient cells. Indeed, siRNA knockdown of Nox1, NOXO1 or Rac1, all components of Nox1-containing NADPH oxidase [21] , in Hace1 −/− MEFs, reversed the increase in ROS to the levels of Hace1 +/+ cells ( Fig. 2b and Supplementary Fig. S3b ). Consistent with this, ROS elevation by independent Hace1 siRNAs in human HEK293 cells (as in Fig. 1d ) was reversed by transient siRNA-mediated co-knockdown of Nox1, NOXA1, NOXO1 or Rac1 ( Fig. 2c and Supplementary Fig. S3c ). Thus, Hace1 inhibits the production of cellular ROS generated by Nox1-containing NADPH oxidase. Next, we analyzed protein levels of known NADPH oxidase subunits in Hace1 −/− versus Hace1 +/+ MEFs. Both cell types displayed equivalent levels of each protein except Rac1, which was markedly elevated in Hace1 −/− MEFs ( Fig. 2d ). Indeed, Rac1 knockdown using independent siRNAs significantly reduced ROS in Hace1 −/− MEFs ( Fig. 2e ), and in human U2OS osteosarcoma cells ( Fig. 2f ). This suggests that elevated ROS in Hace1-deficient cells originates from Rac1-dependent NADPH oxidases. GTP-loaded Rac1, the only known target of the Hace1 E3 ligase, is essential for activation of Nox1, Nox2 and Nox3 containing NADPH oxidases [30] . We therefore investigated whether the mechanism by which Hace1 regulates NADPH oxidase and cellular ROS levels relies on Rac1. GTP-bound Rac1 is ubiquitylated by Hace1 at lysine (K)-147 (ref. 10 ). We therefore analyzed ROS levels in U2OS cells after overexpression of wt Rac1, a constitutively active Rac1-v12, or a Hace1-resistant Rac1-K147R mutant [10] . Both wt Rac1 and the Rac1-v12 mutant significantly increased ROS levels, which could be reversed by either the ML171 NADPH oxidase inhibitor or Hace1 overexpression ( Fig. 2g ). In contrast, ROS levels in cells expressing Hace1-resistant Rac1-K147R were not affected by Hace1 overexpression, indicating that Hace1 must directly target Rac1 to reduce ROS levels. We then tested Hace1 effects in SKOV3 ovarian carcinoma cells, which predominantly express Nox2 rather than Nox1 or Nox3 ( Supplementary Fig. S3d and ref. 31 ). As shown in Fig. 2h , Hace1 also strongly inhibited ROS generation in SKOV3 cells, and siRNAs to Nox2 but not to Nox1 decreases ROS in SKOV3 cells to the same extent as observed with Hace1 overexpression or Rac1 knockdown ( Fig. 2h and Supplementary Fig. S3e,f ). Therefore, Hace1 regulates a second Rac1-dependent complex, namely Nox2-containing NADPH oxidase. Together, these data indicate that Hace1 regulates multiple Rac1-dependent NADPH oxidases by targeting Rac1 for degradation. 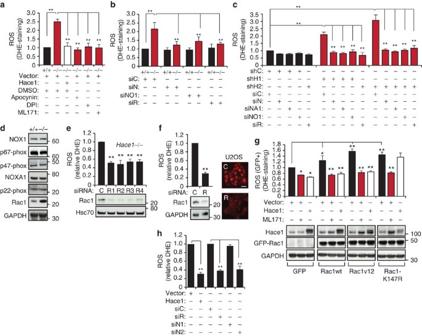Figure 2: Rac1 is required for increased ROS levels in Hace1-deficient cells. (a) MEFs derived from wild-type (+/+) or Hace1 knockout (−/−) mice transfected with HA-vector (Vector) or HA-Hace1 (Hace1) cDNA were left untreated (dimethylsulphoxide) or treated with 5 μM ML171, 5 μM DPI or 400 μM APO before incubated with DHE, analyzed for oxyethidium staining by a 595-nm enabled fluorescence microscope and quantified using ImageJ algorithm. (b) MEFs analogous toatransfected with control (siC), Nox1 (siN), NOXO1 (siNO1) or Rac1 (siR) siRNAs were treated and analyzed as ina. (c) HEK293 cells expressing short hairpin RNA control (shC) or Hace1 (shH1 and shH2) shRNAs and transiently transfected with control (siC), Nox1 (siN), NOXA1 (siNA1), NOXO1 (siNO1) or Rac1 (siR) siRNAs were treated and analyzed as ina. (d) Protein lysates from MEFs derived as inawere analyzed by immunoblotting for the indicated proteins. (e) MEFs derived as inatransfected with control siRNA (C) or siRNAs targeting Rac1 (R1-4) were analyzed for ROS content as ina(graph column) and for expression of the indicated proteins by immunoblotting. (f) U2OS cells were transfected with control siRNA (C) or a siRNA targeting Rac1 (R) before analyzed for ROS content as ina(graph column and sample images) and for expression of the indicated proteins by immunoblotting. Scale bar, 10 μm. (g) U2OS cells transfected with combinations of HA-vector, HA-Hace1, GFP-vector, GFP-Rac1, GFP-Rac1-v12 and GFP-Rac1-K147R and treated with ML171 as indicated, were analyzed for ROS(upper panels) as ina. Protein lysates from the same cells were analyzed for expression of the indicated proteins by immunoblotting (lower). (h) SKOV3 cells were transfected with HA-vector (Vector) or HA-Hace1 (Hace1) cDNA for 48 h, or with control (siC), Nox1 (siN1), Nox2 (siN2) or Rac1 (siR) siRNAs were incubated with DHE and analyzed as ina. For all panels when indicated, *P<0.05; **P<0.01 (Student’s two-tailedt-test for equal variance); Error bars represent s.e.m. of at least three independent experiments. Figure 2: Rac1 is required for increased ROS levels in Hace1-deficient cells. ( a ) MEFs derived from wild-type (+/+) or Hace1 knockout (−/−) mice transfected with HA-vector (Vector) or HA-Hace1 (Hace1) cDNA were left untreated (dimethylsulphoxide) or treated with 5 μM ML171, 5 μM DPI or 400 μM APO before incubated with DHE, analyzed for oxyethidium staining by a 595-nm enabled fluorescence microscope and quantified using ImageJ algorithm. ( b ) MEFs analogous to a transfected with control (siC), Nox1 (siN), NOXO1 (siNO1) or Rac1 (siR) siRNAs were treated and analyzed as in a . ( c ) HEK293 cells expressing short hairpin RNA control (shC) or Hace1 (shH1 and shH2) shRNAs and transiently transfected with control (siC), Nox1 (siN), NOXA1 (siNA1), NOXO1 (siNO1) or Rac1 (siR) siRNAs were treated and analyzed as in a . ( d ) Protein lysates from MEFs derived as in a were analyzed by immunoblotting for the indicated proteins. ( e ) MEFs derived as in a transfected with control siRNA (C) or siRNAs targeting Rac1 (R1-4) were analyzed for ROS content as in a ( graph column ) and for expression of the indicated proteins by immunoblotting. ( f ) U2OS cells were transfected with control siRNA (C) or a siRNA targeting Rac1 (R) before analyzed for ROS content as in a (graph column and sample images) and for expression of the indicated proteins by immunoblotting. Scale bar, 10 μm. ( g ) U2OS cells transfected with combinations of HA-vector, HA-Hace1, GFP-vector, GFP-Rac1, GFP-Rac1-v12 and GFP-Rac1-K147R and treated with ML171 as indicated, were analyzed for ROS (upper panels ) as in a . Protein lysates from the same cells were analyzed for expression of the indicated proteins by immunoblotting ( lower ). ( h ) SKOV3 cells were transfected with HA-vector (Vector) or HA-Hace1 (Hace1) cDNA for 48 h, or with control (siC), Nox1 (siN1), Nox2 (siN2) or Rac1 (siR) siRNAs were incubated with DHE and analyzed as in a . For all panels when indicated, * P <0.05; ** P <0.01 (Student’s two-tailed t -test for equal variance); Error bars represent s.e.m. of at least three independent experiments. Full size image Hace1 targets Rac1 bound to the NADPH oxidase complex As Rac1 is an essential component of Nox1, 2 and 3-containing NADPH oxidase [32] , we hypothesized that Hace1 specifically targets for degradation the fraction of Rac1 that is localized and bound to the holoenzyme. We first confirmed that Rac1 is ubiquitylated by Hace1 in our system by re-expressing Hace1 in Hace1 −/− MEFs ( Fig. 3a ), consistent with previous findings [9] , [10] . As GTP-loaded Rac1 binds NOXA1 at the complex to activate Nox1-containing NADPH oxidase [30] , we tested whether Hace1 also physically associates with NOXA1. Using a green fluorescent protein (GFP)-TRAP pull-down assay, NOXA1 and Rac1 were readily coimmunoprecipitated with GFP-Hace1. Knockdown of Rac1 using siRNAs dramatically inhibited the interaction between NOXA1 and Hace1 ( Fig. 3b ). This indicates that Hace1 binds and targets Rac1 once the latter has been recruited to the complex. To validate this we analyzed whether NOXA1 is required for Rac1 ubiquitylation by Hace1. Indeed, siRNA-mediated NOXA1 knockdown completely blocked Hace1 ubiquitylation of Rac1 ( Fig. 3c ), indicating that Hace1 preferentially targets NOXA1-associated Rac1. Accordingly, the ability of Hace1 to control ROS levels depend on its ligase activity, as expression of a ligase-dead C876S (CS) Hace1 mutant failed to reduce ROS ( Fig. 3d ). To obtain further genetic support for our model, we utilized MEFs derived from mice with targeted deletions of Nox1 ( Nox1 −/− ) or Nox4 ( Nox4 −/− ), as Nox1-containing NADPH oxidase complexes are Rac1-dependent while Nox4-containing complexes are Rac1-independent [32] . While Hace1 knockdown failed to increase ROS in Nox1 −/− MEFs, it markedly did so in wt and Nox4 −/− MEFs ( Fig. 3e ). These findings demonstrate that direct Hace1 targeting of NOXA1-bound Rac1 controls basal ROS levels generated by Rac1-dependent NADPH oxidase complexes. 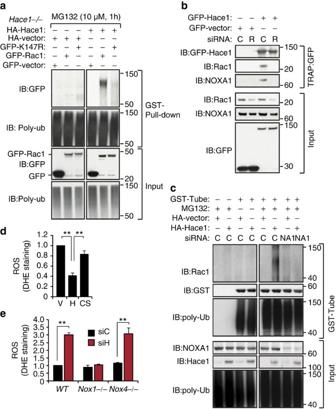Figure 3: Hace1 regulates the Nox1-containing NADPH oxidase. (a) MEFs derived from the Hace1 knockout (−/−) mouse were transfected with HA-vector or HA-Hace1 in denoted combinations of GFP-vector, GFP-Rac1wt and GFP-Rac1-K147R for 48 h before incubated with the proteasome inhibitor MG132 for 2 h, lysed in the presence of GST-TUBE2, subjected a GST pull-down and analyzed by immunoblotting for the indicated proteins. (b) Protein lysates from U2OS cells transfected with siRNA control (C), siRNA Rac1 (R), GFP-vector and GFP-Hace1 as indicated for 72 h, were subjected to GFP:TRAP pull-downs of Hace1 interacting molecules and analyzed by immunoblotting for the indicated proteins. (c) U2OS cells transfected with HA-vector, HA-Hace1 in combinations with control (C) or NOXA1 (NA1) siRNAs for 72 h, were incubated with 10 μM MG132 and lysed with or without GST-TUBE2 as indicated, before being subjected to GST pull-downs and analyzed by immunoblotting for the indicated ubiquitylated proteins. (d) U2OS cells expressing empty vector (V), wild-type Hace1 (H), or C876S ligase-dead Hace1 (CS) were incubated with 10 μM DHE for 30 min, analyzed for oxyethidium stainingby a 595-nm enabled fluorescence microscope and quantified using ImageJ algorithm. (e) MEFs derived from wild-type (wt), Nox1-deficient (Nox1−/−) and Nox4-deficient (Nox4−/−) mice, were transfected with control (siC) or Hace1 (siH) siRNAs 72 hrs before being analyzed for ROS content as inc. For all panels when indicated, **P<0.01 (Student’s two-tailedt-test for equal variance); Error bars represent s.e.m. of at least three independent experiments. Figure 3: Hace1 regulates the Nox1-containing NADPH oxidase. ( a ) MEFs derived from the Hace1 knockout (−/−) mouse were transfected with HA-vector or HA-Hace1 in denoted combinations of GFP-vector, GFP-Rac1wt and GFP-Rac1-K147R for 48 h before incubated with the proteasome inhibitor MG132 for 2 h, lysed in the presence of GST-TUBE2, subjected a GST pull-down and analyzed by immunoblotting for the indicated proteins. ( b ) Protein lysates from U2OS cells transfected with siRNA control (C), siRNA Rac1 (R), GFP-vector and GFP-Hace1 as indicated for 72 h, were subjected to GFP:TRAP pull-downs of Hace1 interacting molecules and analyzed by immunoblotting for the indicated proteins. ( c ) U2OS cells transfected with HA-vector, HA-Hace1 in combinations with control (C) or NOXA1 (NA1) siRNAs for 72 h, were incubated with 10 μM MG132 and lysed with or without GST-TUBE2 as indicated, before being subjected to GST pull-downs and analyzed by immunoblotting for the indicated ubiquitylated proteins. ( d ) U2OS cells expressing empty vector (V), wild-type Hace1 (H), or C876S ligase-dead Hace1 (CS) were incubated with 10 μM DHE for 30 min, analyzed for oxyethidium stainingby a 595-nm enabled fluorescence microscope and quantified using ImageJ algorithm. ( e ) MEFs derived from wild-type (wt), Nox1-deficient (Nox1−/−) and Nox4-deficient (Nox4−/−) mice, were transfected with control (siC) or Hace1 (siH) siRNAs 72 hrs before being analyzed for ROS content as in c . For all panels when indicated, ** P <0.01 (Student’s two-tailed t -test for equal variance); Error bars represent s.e.m. of at least three independent experiments. Full size image Hace1 deficiency leads to NADPH oxidase-dependent DNA damage We next wished to determine the physiological consequences of NADPH oxidase regulation by Hace1. As Hace1 −/− mice are prone to tumorigenesis after IR or urethane treatment [6] , both of which induce DNA damage through ROS generation, we postulated that chronic elevated NADPH oxidase-mediated ROS might lead to increased DNA damage in Hace1-deficient cells. ROS-induced DNA damage response depends on ataxia-telangiectasia mutated (ATM) and the tumor suppressor p53, which are both phosphorylated in their active forms after DNA damage [33] , [34] . Exposure of Hace1 −/− MEFs to low concentrations of exogenous H 2 O 2 to simulate DNA damage markedly increased ATM and p53 Ser-15 phosphorylation compared with Hace1 +/+ cells, each of which was reduced by transient re-expression of wt Hace1 ( Fig. 4a ; see GFP-Hace1 lanes). Low-dose IR also led to markedly higher phosphorylation of histone H2AX on serine 139 (γH2AX), another well-established readout of DNA damage [35] , in Hace1 −/− versus Hace1 +/+ MEFs ( Fig. 4b ), which again was reversed by transient wt Hace1 re-expression in the former ( Fig. 4d ). The difference in γH2AX levels between Hace1 −/− versus Hace1 +/+ MEFs was already observed after 5 min of recovery from low-dose IR ( Supplementary Fig. S3g ), suggesting that this response is due to acute ROS generated by IR [36] . However, we cannot rule out whether DNA damage induced ROS amplification through other mechanisms, such as by direct H2AX activation of Nox1 [37] may amplify the system. Similarly, in U2OS cells, exogenous H 2 O 2 -mediated ATM and γH2AX phosphorylation was blocked by transient Hace1 overexpression ( Fig. 4e ), which reduces ROS in those cells ( Fig. 2f ). We then tested whether increased susceptibility to ROS-induced DNA damage in Hace1-deficient cells is dependent on Nox1-containing NADPH oxidase. Indeed, in Hace1 −/− MEFs, ML171 blocked H 2 O 2 -induced ATM phosphorylation ( Fig. 4f ) and Nox1 knockdown blocked exogenous H 2 O 2 -induced p53 Ser-15 phosphorylation ( Fig. 4g ). Moreover, while Hace1 knockdown sensitized wt MEFs to H 2 O 2 -induced DNA damage, this was almost completely blocked in Nox1 −/− MEFs exposed to H 2 O 2 ( Fig. 4h ). Therefore, augmented DNA damage responses secondary to Hace1 deficiency require Rac1-dependent NADPH oxidase activity. Finally, the human breast carcinoma cell line HCC1395, which lacks Hace1 expression due to a homozygous deletion of HACE1 , had dramatically elevated γH2AX phosphorylation levels compared with HEK293 cells, even under ambient conditions ( Fig. 4i ). Finally, hace1 morpholino zebrafish showed a striking increase in γH2AX phosphorylation under basal conditions compared with wt fish ( Fig. 4j ). These data provide compelling evidence that Hace1 -deficient cells are hypersensitive to ROS-induced DNA damage. 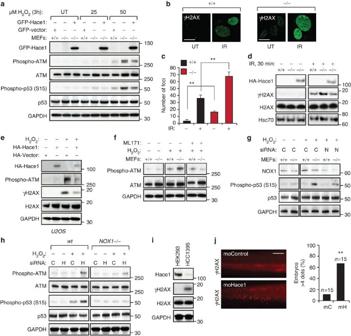Figure 4: Loss of Hace1 leads to Nox1-dependent activation of the DNA damage response. (a) MEFs derived from wild-type (+/+) or Hace1 knockout (−/−) mice were transfected with GFP-vector or GFP-Hace1 48 h before being untreated (UT) or treated with indicated concentrations of H2O2for 3 h and analyzed by immunoblotting for the indicated proteins. (b) MEFs derived as inawere subjected to 6 Gy IR for 1 h as indicated and analyzed for phosphorylated histone H2AX (γH2AX) by immunostaining. Scale bar, 5 μm. (c) Quantification of γH2AX foci formation in high-power images obtained as inb. (d) Lysates obtained from MEFs treated as inbwere analyzed for expression of the indicated proteins by immunoblotting. (e) U2OS osteosarcoma cells transfected with HA-vector or HA-Hace1 for 48 h were left untreated or treated with 400 μM H2O2for 3 h before being analyzed by immunoblotting for the indicated proteins. (f) MEFs derived as inawere treated with 10 μM ML171 or 50 μM H2O2as indicated and analyzed by immunoblotting for the indicated proteins. (g) MEFs derived as inawere transfected with control (C) or Nox1 (N) siRNAs, and treated with 50 μM H2O2as indicated for 3 h and analyzed by immunoblotting for the indicated proteins. (h) MEFs derived from wild-type (wt) or Nox1 knockout (Nox1−/−) mice were transfected with control (C) or Hace1 (H) siRNAs, treated with 50 μM H2O2as indicated for 3 h and analyzed by immunoblotting for the indicated proteins. (i) HEK293 human embryonic kidney cells and HCC1395 breast cancer cells deficient for Hace1 expression were analyzed for phosphorylated histone H2AX (γH2AX) by immunoblotting. (j) Representative images (left) of 48 h post fertilization (hpf) casper zebrafish control (mC) and hace1 (mH) morphants stained for phosphorylated histone H2AX (γH2AX). The column graph (right) displays % embryos (n=15) with more than four γH2AX dots per tail. Scale bar, 0.25 mm. For all panels when indicated, **P<0.01 (Student’s two-tailedt-test for equal variance); Error bars represent s.e.m. of at least three independent experiments. Figure 4: Loss of Hace1 leads to Nox1-dependent activation of the DNA damage response. ( a ) MEFs derived from wild-type (+/+) or Hace1 knockout (−/−) mice were transfected with GFP-vector or GFP-Hace1 48 h before being untreated (UT) or treated with indicated concentrations of H 2 O 2 for 3 h and analyzed by immunoblotting for the indicated proteins. ( b ) MEFs derived as in a were subjected to 6 Gy IR for 1 h as indicated and analyzed for phosphorylated histone H2AX (γH2AX) by immunostaining. Scale bar, 5 μm. ( c ) Quantification of γH2AX foci formation in high-power images obtained as in b . ( d ) Lysates obtained from MEFs treated as in b were analyzed for expression of the indicated proteins by immunoblotting. ( e ) U2OS osteosarcoma cells transfected with HA-vector or HA-Hace1 for 48 h were left untreated or treated with 400 μM H 2 O 2 for 3 h before being analyzed by immunoblotting for the indicated proteins. ( f ) MEFs derived as in a were treated with 10 μM ML171 or 50 μM H 2 O 2 as indicated and analyzed by immunoblotting for the indicated proteins. ( g ) MEFs derived as in a were transfected with control (C) or Nox1 (N) siRNAs, and treated with 50 μM H 2 O 2 as indicated for 3 h and analyzed by immunoblotting for the indicated proteins. ( h ) MEFs derived from wild-type ( wt ) or Nox1 knockout ( Nox1 −/− ) mice were transfected with control (C) or Hace1 (H) siRNAs, treated with 50 μM H 2 O 2 as indicated for 3 h and analyzed by immunoblotting for the indicated proteins. ( i ) HEK293 human embryonic kidney cells and HCC1395 breast cancer cells deficient for Hace1 expression were analyzed for phosphorylated histone H2AX (γH2AX) by immunoblotting. ( j ) Representative images ( left ) of 48 h post fertilization (hpf) casper zebrafish control ( mC ) and hace1 ( mH ) morphants stained for phosphorylated histone H2AX (γH2AX). The column graph ( right ) displays % embryos ( n =15) with more than four γH2AX dots per tail. Scale bar, 0.25 mm. For all panels when indicated, ** P <0.01 (Student’s two-tailed t -test for equal variance); Error bars represent s.e.m. of at least three independent experiments. Full size image Hace1 controls cyclin D1 via regulation of ROS production We previously showed that Hace1 reduces in vitro and in vivo cell cycle progression of diverse Hace1 -deficient tumor cell lines by repressing cyclin D1 protein expression, although Hace1 does not directly target cyclin D1 for degradation [6] . We therefore wondered if Hace1 might also control cyclin D1 expression through its effects on Rac1-dependent NADPH oxidases, particularly as induction of CCND1 ( cyclin D1 ) messenger RNA (mRNA) expression has been linked to NADPH oxidase activity [38] . We first investigated Hace1 regulation of ROS after mitogenic stimulation. Serum-starved Hace1 − / − MEFs displayed increased ROS compared with Hace1 +/+ MEFs, and Hace1 − / − cells maintained elevated ROS accumulation in a time-dependent manner after serum re-stimulation ( Supplementary Fig. S4a ). This suggests that Hace1 − / − controls ROS generation even under mitogenic stimulation and that reduced ROS in Hace1 proficient cells is not simply a direct effect of decreased cell proliferation. Indeed, cyclin D1 levels were dramatically increased in Hace1 −/− compared with Hace1 +/+ MEFs and this was inhibited by ML171 or APO ( Fig. 5a ). Moreover, ectopic Hace1 expression reduced cyclin D1 levels in Hace1 −/− MEFs, which was further reduced by ML171 ( Fig. 5b ). Similarly, both Hace1 overexpression ( Fig. 5c ) and Rac1 siRNA knockdown ( Fig. 5d ) strongly reduced cyclin D1 expression in U2OS cells. Overexpression of the Rac1-K147R mutant in these cells upregulated cyclin D1, which was reversed by ML171 ( Fig. 5e ). We then knocked down Hace1 in wt , Nox1 −/− and Nox4 −/− MEFs; this increased cyclin D1 levels in wt and Nox4 −/− MEFs, but failed to do so in Nox1 −/− MEFs ( Fig. 5f ). Therefore, Hace1-deficient cells require Rac1-dependent NADPH oxidase activity to induce cyclin D1 expression. We next analyzed ROS, Rac1 and cyclin D1 levels in a panel of Hace1-deficient human epithelial cancer cell lines ( Fig. 5g ). All cell lines displayed varying but significant increases in ROS, and this correlated strongly with elevated Rac1 and cyclin D1 levels compared with HEK293 cells (which express high Hace1 levels [6] ). Of note, Hace1 mRNA and protein levels both increase in U2OS cells after acute ROS challenge with H 2 O 2 , and this correlates with increased binding and ubiquitylation of Rac1 by Hace1 ( Supplementary Fig. S4b–e ). Hace1 appears to bind only a small fraction of the total Rac1 pool, estimated to be <10% ( Supplementary Fig. S4f ). This suggests that Hace1 expression and protein activity can be amplified by a ROS-dependent activation step to mediate its effect on Rac1 at membrane-associated NADPH oxidase complexes, and therefore on cyclin D1 expression. 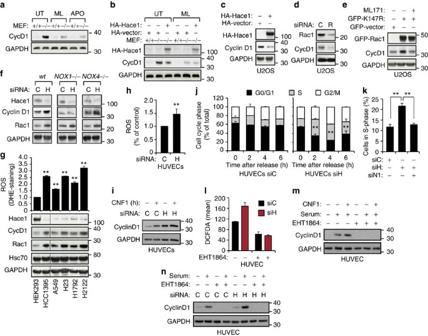Figure 5: Hace1 controls cyclin D1 expression by regulating of Nox1-containing NADPH oxidase. (a) Protein lysates from Hace1 wild-type (+/+) or knockout (−/−) MEFs were left untreated or treated overnight with ML171 (ML) or APO, were analyzed by immunoblotting as indicated. (b) MEFs as inawere transfected with Ha-vector or HA-Hace1, left untreated (UT) or treated overnight with ML171 (ML), and analyzed as ina. (c) U2OS cells transfected with HA-vector or HA-Hace1 were analyzed as ina. (d) U2OS cells transfected with control (C) or Rac1 (R) siRNAs were analyzed as ina. (e) U2OS cells transfected with GFP-vector or GFP-Rac1-K147R were left untreated or treated with ML171, and analyzed as ina. (f) Wild-type (WT),NOX4knockout (NOX4−/−) or NOX1 knockout (NOX1−/−) MEFs were transfected with control (siC) or Hace1 (siH) siRNAs and analyzed as ina. (g) Indicated cell lines were analyzed for ROS by DHE staining and by immunoblotting of indicated proteins. (h) HUVEC cells were transfected with siRNA control (C) or Hace1 (H) and analyzed for ROS content by DCFDA assay. (i) HUVEC cells transfected as inhwere analyzed for the indicated proteins by immunoblotting after stimulation with vehicle or CNF1 (10−9M). (j) HUVEC cells transfected as inhwere analyzed for cell cycle distribution (G1, S, G2/M phase) after release from a thymidine cell cycle block at the indicated time points. (k) HUVEC cells transfected with siRNA control (C), Hace1 (H) or Nox1 (N1) as inhwere analyzed for cells in S-phase after release from a thymidine cell cycle block. (l) HUVEC cells transfected with siRNA control (siC) or Hace1 (siH) were stimulated as ini, treated with EHT1864 as indicated and analyzed for ROS content as inh. (m) Lysates from HUVEC cells synchronized in G0 by serum deprivation and stimulated with serum for 15 h with or without EHT1864 and stimulation with vehicle or CNF1 were analyzed as ina. (n) Lysates from control (C) or HACE1 (H) knocked down HUVEC cells treated as inmwere analyzed as ina. For all panels when indicated, **P<0.01 (Student’s two-tailedt-test); Error bars: s.e.m. of at least three independent experiments. Figure 5: Hace1 controls cyclin D1 expression by regulating of Nox1-containing NADPH oxidase. ( a ) Protein lysates from Hace1 wild-type (+/+) or knockout (−/−) MEFs were left untreated or treated overnight with ML171 (ML) or APO, were analyzed by immunoblotting as indicated. ( b ) MEFs as in a were transfected with Ha-vector or HA-Hace1, left untreated (UT) or treated overnight with ML171 (ML), and analyzed as in a . ( c ) U2OS cells transfected with HA-vector or HA-Hace1 were analyzed as in a . ( d ) U2OS cells transfected with control (C) or Rac1 (R) siRNAs were analyzed as in a . ( e ) U2OS cells transfected with GFP-vector or GFP-Rac1-K147R were left untreated or treated with ML171, and analyzed as in a . ( f ) Wild-type ( WT ), NOX4 knockout ( NOX4 −/−) or NOX1 knockout ( NOX1 −/−) MEFs were transfected with control (siC) or Hace1 (siH) siRNAs and analyzed as in a . ( g ) Indicated cell lines were analyzed for ROS by DHE staining and by immunoblotting of indicated proteins. ( h ) HUVEC cells were transfected with siRNA control (C) or Hace1 (H) and analyzed for ROS content by DCFDA assay. ( i ) HUVEC cells transfected as in h were analyzed for the indicated proteins by immunoblotting after stimulation with vehicle or CNF1 (10 − 9 M). ( j ) HUVEC cells transfected as in h were analyzed for cell cycle distribution (G1, S, G2/M phase) after release from a thymidine cell cycle block at the indicated time points. ( k ) HUVEC cells transfected with siRNA control (C), Hace1 (H) or Nox1 (N1) as in h were analyzed for cells in S-phase after release from a thymidine cell cycle block. ( l ) HUVEC cells transfected with siRNA control (siC) or Hace1 (siH) were stimulated as in i , treated with EHT1864 as indicated and analyzed for ROS content as in h . ( m ) Lysates from HUVEC cells synchronized in G0 by serum deprivation and stimulated with serum for 15 h with or without EHT1864 and stimulation with vehicle or CNF1 were analyzed as in a . ( n ) Lysates from control (C) or HACE1 (H) knocked down HUVEC cells treated as in m were analyzed as in a . For all panels when indicated, ** P <0.01 (Student’s two-tailed t -test); Error bars: s.e.m. of at least three independent experiments. Full size image Lastly, to test whether Hace1 can block cell cycle progression in primary human cells through ROS regulation, freshly isolated human vein endothelial cells (HUVECs) were transfected with control or Hace1 siRNAs and analyzed for ROS content. Hace1 knockdown markedly increased ROS levels in HUVECs as measured by DCFDA staining ( Fig. 5h ). Moreover, while the CNF1 Escherichia coli toxin, which activates Rac1 in HUVECs [9] , could induce cyclin D1 expression in these cells, cyclin D1 was constitutively induced in Hace1 knockdown HUVECs even in the absence of CNF1 ( Fig. 5i ). Importantly, Hace1 knockdown correlated with increased S and G2M fractions and cell proliferation of primary HUVECs ( Fig. 5j ), and co-knockdown of Nox1 decreased the fraction of cells in S-phase to control levels ( Fig. 5k ). Furthermore, the chemical Rac1 inhibitor EHT1864 efficiently reduced ROS in HUVECs with Hace1 knockdown ( Fig. 5l ) and abolished cyclin D1 induction by CNF1 or serum ( Fig. 5m ). Finally, EHT1864 blocked serum-stimulated cyclin D1 induction in HUVECs with Hace1 knockdown ( Fig. 5n ). Collectively, these data suggest that Hace1 controls cyclin D1 expression and cell cycle progression through its ability to block activity of Rac1-dependent NADPH oxidase complexes. Increased ROS in Hace1-deficient murine and human tumors To demonstrate the in vivo significance of the above findings, we examined tissues from Hace1 −/− mice, which develop diverse spontaneous late-onset tumors across all three germ layers [6] . Liver tumors from these mice showed strikingly higher ROS levels than matching normal liver tissue from the same mice, or from Hace1 +/+ littermates ( Fig. 6a ). Hace1 loss strongly correlated with elevated Rac1, cyclin D1 and phosphorylated Ser-15-p53 levels in tumor lysates ( Fig. 6b ). This was also observed in Hace1 −/− mouse colorectal carcinoma as compared to normal tissue ( Fig. 6c ). This indicates that not only do normal tissues of Hace1 −/− mice have higher ROS levels compared with wt mice ( Fig. 1e ), but there is further ROS accumulation in the tumors, possibly due to clonal selection during transformation. As Hace1 was originally discovered as a tumor suppressor in human Wilms’ tumor [1] , [6] , we next investigated a panel of patient-matched Wilms’ tumor and normal kidney specimens, each previously documented to have lost Hace1 protein expression [1] . All tumors analyzed displayed markedly increased ROS ( Fig. 6d ), which correlated with elevated Rac1 and cyclin D1 expression, as well as phosphorylated Ser-15-p53 levels ( Fig. 6f ). This clearly demonstrates that Hace1-deficient mouse and human tumors have chronic high ROS, elevated Rac1 and cyclin D1 expression, which is coupled with increased DNA damage response signaling, confirming the in vivo significance of our findings. 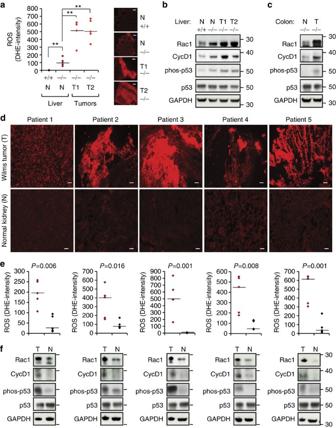Figure 6: Characterization of murine and human Hace1-deficient tumors. (a) Snap-frozen samples of normal liver (N) fromwild-type(+/+) andHace1−/− mice (−/−) and matching spontaneous liver tumor tissues (T1 and T2) from the sameHace1−/− mice were cut in 20 μm sections using a cryostat at −20 °C, incubated with 10 μM DHE for 30 min and analyzed for oxyethidium staining by a 595-nm enabled fluorescence microscope (right) and quantified using ImageJ algorithm (left). Scale bars, 20 μm. Horizontal lines in the graphs represent median values of quantification by ImageJ algorithm. **P>0.01 (Student’s two-tailedt-test for equal variance). (b) Protein lysates isolated from tissues shown inawere analyzed for expression levels of the indicated proteins by immunoblotting. (c) Protein lysates from normal colon tissue (N) and colonic tumor tissue (T) dissected from Hace1 knockout (−/−) mice were analyzed for the expression of the indicated proteins by immunoblotting. (d) Snap-frozen tissue of matched normal kidney (N) and Wilms’ tumors (T) from the same patients were analyzed for ROS as ina. Scale bars, 20 μm. (e) High power field images obtained as indwere quantified for DHE signal intensity (ROS content) by ImageJ software. Lines represent median values. (f) Lysates from tissue as indwere analyzed for expression of the indicated proteins (lower panels) by immunoblotting. Figure 6: Characterization of murine and human Hace1-deficient tumors. ( a ) Snap-frozen samples of normal liver (N) from wild-type (+/+) and Hace1 −/− mice (−/−) and matching spontaneous liver tumor tissues (T1 and T2) from the same Hace1 −/− mice were cut in 20 μm sections using a cryostat at −20 °C, incubated with 10 μM DHE for 30 min and analyzed for oxyethidium staining by a 595-nm enabled fluorescence microscope ( right ) and quantified using ImageJ algorithm ( left ). Scale bars, 20 μm. Horizontal lines in the graphs represent median values of quantification by ImageJ algorithm. ** P >0.01 (Student’s two-tailed t -test for equal variance). ( b ) Protein lysates isolated from tissues shown in a were analyzed for expression levels of the indicated proteins by immunoblotting. ( c ) Protein lysates from normal colon tissue (N) and colonic tumor tissue (T) dissected from Hace1 knockout (−/−) mice were analyzed for the expression of the indicated proteins by immunoblotting. ( d ) Snap-frozen tissue of matched normal kidney (N) and Wilms’ tumors (T) from the same patients were analyzed for ROS as in a . Scale bars, 20 μm. ( e ) High power field images obtained as in d were quantified for DHE signal intensity (ROS content) by ImageJ software. Lines represent median values. ( f ) Lysates from tissue as in d were analyzed for expression of the indicated proteins ( lower panels ) by immunoblotting. Full size image ROS are essential for cell homeostasis and has diverse roles in health and disease. Along with the mitochondria, which continuously generate ROS as byproducts of oxidative phosphorylation [39] , a major source of cellular ROS are the NADPH oxidases [21] . These enzymes utilize molecular oxygen and NADPH to produce superoxide, which is then rapidly converted to cellular H 2 O 2 by superoxide dismutase enzymes [21] . NADPH oxidase complexes are found in all multicellular organisms where they are solely dedicated to the generation of ROS. In non-pathological settings, ROS functions as a second messenger for processes such as differentiation, proliferation and cell motility [40] . In pathologic conditions, however, ROS can oxidize biomolecules such as DNA, causing DNA damage and is likely the greatest intrinsic threat to genome integrity. Accordingly, organisms have evolved a tightly regulated cellular response to acute oxidative stress to detoxify ROS and repair damaged DNA [33] . While cellular detoxification systems are well-characterized [41] , little is known about the regulation of ROS generation by NADPH oxidases. Here we identify the tumor suppressor Hace1 as a highly conserved direct negative regulator of Rac1-dependent NADPH oxidases through degradation of complex-bound Rac1. Hace1 deficiency leads to a deregulated and hyperactive ROS-generating holoenzyme that maintains a state of chronic high ROS in vitro and in vivo . This is associated with ROS-induced DNA damage and cyclin D1 expression, both of which are blocked by pharmacologic or genetic inactivation of Nox1-containing NADPH oxidases. Based on these observations, we propose a model whereby Hace1 recruitment to Rac1-containing NADPH oxidases leads to Rac1 degradation and inactivation of the complex ( Fig. 7 ). Together with Rac1 guanine nucleotide exchange-factors [42] , Hace1-mediated ubiquitylation of Rac1 therefore adds another layer of control to the regulation of the NADPH oxidase system. These results highlight a novel regulatory pathway that protects cells from ROS-induced DNA damage and cyclin D1-mediated hyperproliferation. This is the first known example, to our knowledge, of an E3 ligase that directly regulates NADPH oxidase activity and of a tumor suppressor that directly regulates ROS generation in vertebrate cells. 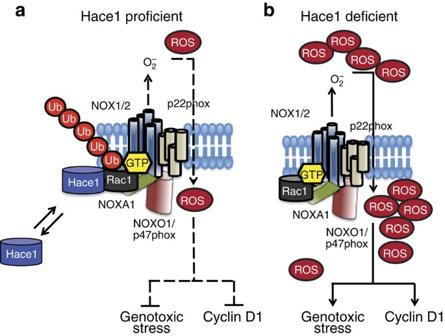Figure 7: Hace1 controls NADPH oxidase. (a) Hace1 targets complex-bound Rac1 to regulate NADPH oxidase, ROS production, cyclin D1 expression and DNA damage susceptibility. (b) Loss of Hace1 leads to hyperactive NADPH oxidase activity, increased ROS generation, high cyclin D1 expression and ROS-induced DNA damage. Figure 7: Hace1 controls NADPH oxidase. ( a ) Hace1 targets complex-bound Rac1 to regulate NADPH oxidase, ROS production, cyclin D1 expression and DNA damage susceptibility. ( b ) Loss of Hace1 leads to hyperactive NADPH oxidase activity, increased ROS generation, high cyclin D1 expression and ROS-induced DNA damage. Full size image Activation of Rac1-dependent NADPH oxidase complexes requires the binding of GTP-loaded Rac1 to the NADPH oxidase subunit, Noxa1. Mechanistically, we show that Hace1 binds and ubiquitinates Rac1 when the latter associates with the complex through Noxa1. This then targets complex-bound Rac1 for proteasomal degradation and inhibits NADPH oxidase activity. Whether Hace1 requires an activation step before it can bind Rac1 at the complex is currently unknown. HACE1 has recently been implicated as a target gene of the Nrf2 transcription factor [43] . Nrf2 regulates transcription of a wide spectrum of genes involved in the oxidative stress response [43] . Indeed, Hace1 mRNA and protein levels are increased in U2OS cells after acute ROS challenge with H 2 O 2 . It is therefore tempting to speculate that Hace1 becomes activated by oxidative stress to subsequently shut down one of the main ROS-generating enzymes in cells as a part of the general oxidative stress response. While somewhat contentious, the current view is that Nox1, Nox2 and Nox3 containing NADPH oxidase complexes are clearly Rac1-dependent for activation, while Nox4, Nox5 and DUOX containing complexes are Rac1-independent [21] , [44] . Nox1 is thought to be the major Nox subunit of NADPH oxidases in epithelial and mesenchymal cells, while Nox2 expression is more restricted to hematopoietic cells [21] . However, Nox2 may have broader expression in epithelial and mesenchymal cells, while Nox3 is expressed only at low levels in these cell types (ref. 31 ). Our studies point to a general role for Hace1 in regulating Rac1-containing NADPH oxidase complexes as it blocks ROS generated from both Nox1- and Nox2-containing complexes. As Hace1 only binds a small fraction of the total Rac1 pool, estimated as <10% and mainly associated with NADPH oxidase, it is unknown whether Hace1 targets other subcellular pools of GTP-Rac1 under context-specific conditions. Ros can be pro-oncogenic as a consequence of increased replication stress and incomplete repair of ROS-induced DNA damage. Rac1 and Nox1 are required for cellular transformation by numerous oncogenes including activated K-Ras, H-Ras, c-Met, c-Myc and c-Src, and oncogene transformation is consistently associated with elevated ROS levels [45] , [46] , [47] , [48] , [49] . While the role of ROS in transformation is incompletely understood, elevated ROS produced by oncogenic signaling may contribute to the accumulation of additional mutations, further supporting tumor progression. Disruption of the Hace1-Rac1-NADPH oxidase axis described here may therefore impact a potentially broad spectrum of human tumors. As ROS scavenging by anti-oxidants inhibits the transformed phenotype [50] , transformed cells may become addicted to chronic high ROS levels to maintain specific aspects of pro-oncogenic signaling. Interestingly, induction of CCND1 ( cyclin D1 ) mRNA expression by the AP-1 transcription factor is known to require NADPH oxidase activity [38] . Indeed, we demonstrate that cyclin D1 induction in Hace1-deficient cells also depends on intact Rac1 and NADPH oxidase activity. D-type cyclins (D1 and D3 in particular) have recently been linked to the maintenance of tumor growth in both epithelial and hematopoietic malignancies [51] , [52] . Therefore, the NADPH oxidase and ROS-driven cyclin D1 expression observed in Hace1-deficient cells might contribute broadly to progression of spontaneous tumors. We found that the EHT1864 Rac1 inhibitor strongly blocks ROS-induced cyclin D1 expression, a finding that may have clinical implications. Also, as ROS has pathogenic roles in other human diseases such as cardiac hypertrophy and ischemia-reperfusion injury, immune system disorders, liver disease, diabetes, obesity, atherosclerosis, Alzheimer’s disease, Parkinson’s disease, Huntington disease, rheumatoid arthritis, aging and HIF1/hypoxia-related diseases [53] , [54] , [55] , [56] , further studies of pathogenic Hace1 deficiency may reveal additional disease links. In summary, we find that Hace1 deficiency leads to chronic elevated cellular ROS and ROS-induced DNA damage response signaling, which is blocked by pharmacologic or genetic inactivation of Rac1-containing NADPH oxidases. These results identify Hace1 as a de facto negative regulator of NADPH oxidase activity in vertebrates and highlight a novel regulatory pathway that protects cells from ROS-induced DNA damage. It will be important to determine how this specific function of Hace1 contributes to its tumor suppressor activity, and whether Hace1 deficiency has roles in other pathologic conditions. Cell culture and reagents All cells were grown in DMEM (Dulbecco) supplemented with 10% fetal calf serum, non-essential amino acids and penicillin–streptomycin. Wild-type ( wt ) and Hace1 knockout MEFs were derived from BL6 WT and Hace1−/− littermates and allowed to spontaneously immortalize. WT, Nox1 −/− and Nox4 −/− MEFs were a kind gift from Dr Denis Martinvalet, University of Geneva. HUVEC cells were derived as described in Torrino et al . [9] . DNA transfections were performed with FugeneHD for human cell lines and with electroporation using Neon Transfection System (Invitrogen) for mouse cell lines. MSCV-HA, MSCV-HA-Hace1 and MSCV-HA-Hace1-C876S were cloned as described in Zhang et al . [6] . GFP-Hace1 and GFP Hace1-C876S were generated by cloning Hace1 and C876S into pEGFP-C1 (Clontech). GFP-Rac1wt, GFP-Rac-1v12 were generated as described in Castillo-Lluva et al . [57] and GFP-Rac1-K147R was made by PCR-based nucleotide mutagenesis in GFP-Rac1. Transfections of siRNAs were performed with 25 nM siRNA using RNAiMax (Invitrogen). The following siRNAs were used in the study: Control siRNA (C): (5′–3′) AUAUCGGCUAGGUCUAACA; Hace1-1 (H1): Hs_Hace1_1 (FlexiTube, Qiagen); Hace1-2 (H2): Hs_Hace1_4 (FlexiTube, Qiagen); Human Rac1 (R): Hs_Rac1_6 (FlexiTube, Qiagen); Human Nox2 (N2): Hs_CYBB (FlexiTube, Qiagen); Murine Rac1-1 (R1): Mm_Rac1_1 (FlexiTube, Qiagen); Murine Rac1-2 (R2): Mm_Rac1_2 (FlexiTube, Qiagen); Murine Rac1-3 (R3): Mm_Rac1_3 (FlexiTube, Qiagen); Murine Rac1-4 (R4): Mm_Rac1_8 (FlexiTube, Qiagen). Human and mouse Nox1, human NoxA1, human and mouse NOXO1 and mouse p22phox siRNA ON-TARGETplus SMARTpools were obtained from Dharmacon. Camptothecin, hydrogen peroxide (H 2 O 2 ), DPI, 2-acetylphenothiazine (ML171), APO, DHE, EHT1864 and MG132 were purchased from Sigma. Piperlongumine (PL) was purchased from RD Chemicals. IR was performed in an X-ray generator (Pantak HF160, 150 kV, 15 mA, dose rate 2.18 Gy per minute). Reactive oxygen species measurements Crude ROS levels were measured by CM-H2-DCFDA (Invitrogen) according to the manufacturer’s guidelines. Primary cells (HUVECs) were incubated with 5 mM 2',7'-dichlorodihydrofluorescein diacetate (DCFDA, Santa-Cruz) for 20 min at 37 °C. Cells were washed twice in PBS, trypsinized and fluorescence was measured using flow cytometry. For each experiment, fluorescence was determined on triplicate samples. Statistical analysis of the results was performed with Prism 5.0b (GraphPad software) by one-way ANOVA with Bonferroni post hoc . Superoxide levels were measured using the DHE probe. In the presence of the superoxide anion O 2 − , DHE is rapidly oxidized to oxyethidium, which binds DNA and emits light in the 570–580 nm ranges when excited at 488 nm. For cell culture, after appropriate treatments, cells were washed in Hank’s Balanced Salt Solution (HBSS), incubated for 30–60 min in HBSS containing 10 μM DHE, washed in HBSS and directly analyzed for oxyethidium fluorescence with an epi-fluorescence HAL100 microscope (Zeiss). For tissue sections, snap-frozen tissue samples and tumors were cut in 20 μm sections using a cryostat, washed and DHE-treated as described for cell lines, mounted on cover slides and analyzed as for cell lines. When indicated, oxyethidium emission was analyzed and quantified using ImageJ software. For all specimens, haematoxylin and eosin staining were performed side-by-side to verify tissue integrity and pathology, using standard methods. NTB was used to detect localized ROS in vitro . When NTB becomes oxidized it creates an insoluble blue formazan dye detectable using a high-resolution light microscope. Exponentially growing cells were incubated with a saturated NTB solution (in H 2 O) for 30 min in 37 °C before washed 2 × in PBS, air-dried and analyzed in a 60 × magnification light microscope. Immunodetection For immunoblotting, proteins separated by SDS–polyacrylamide gel electrophoresis (PAGE) and transferred to a nitrocellulose membrane were detected with indicated primary and appropriate secondary antibodies, enhanced chemiluminescence (ECL) western blotting reagents (Thermo Scientific), and film (Kodak). Primary antibodies used in the indicated dilutions were purchased from Sigma (Hace1 (1:1,000), NOXA1 (1:500), Nox1 (1:300), Roche (GFP (1:2,000)), Rockland (phospho-S1981-ATM (1:1,000)), Cell Signaling (ATM (1:1,000), p53 (1:1,000), phosphoS15-p53 (1:1,000), phosphoS139-H2AX (1:1,000), H2AX (1:1,000), GAPDH (1:2,000), cyclin D1 (1:1,000)), BD Biosciences (Rac1 (1:500)), Santa-Cruz (Rac1 (1:1,000), p22phox (1:250), p67phox (1:500), p47phox (1:500), GST (1:1,000), Nox2 (1:500)), ENZO (poly-ubiquitin (1:1,000)), Assay Designs (Hsc70 (1:1,000)) and Covance (HA (1:1,000)). Secondary horseradish peroxidase-conjugated antibodies (1:10.000) used for immunoblotting were purchased from DAKO. Full-length scans of immunoblots with key data are shown in Supplementary Fig. S5 . GFP:TRAP and TUBE pull-down assays For GFP:TRAP pull-downs, whole-cell lysates were dissolved in TRAP-buffer (10 mM Tris-HCL pH 7.5, 0.5% NP-40, 150 mM NaCl, 0.5 mM EDTA) supplemented with 1 nM PMSF (Active Motif) protease and phosphatase inhibitors (Roche). Clarified extracts were incubated for 3 h in a rotator at 4° C with 30 μl GFP-Trap_A beads (Chromotech). Precipitated immunocomplexes were washed 5 × in TRAP-buffer without NP-40, boiled in SDS sample buffer containing 50 mM dithiothreitol, and analyzed by immunoblotting. TUBEs were used to purify endogenous ubiquitin conjugates from cell lysates according to the manufacturer’s recommendations with minor modifications. Briefly, lysis buffer (20 mM Na 2 HPO 4 , 20 mM NaH 2 PO 4 , 1% NP-40, 2 mM EDTA) was supplemented with 1 mM dithiothreitol, 1 × protease inhibitor mix (Sigma) and 50 μg ml −1 of GST-TUBE2 (Lifesensors, Malvern, PA). One 70–80% confluent 10 cm dish per condition was treated as indicated, after which cells were scraped off the dish in PBS and pelleted by centrifugation. Cells were lysed in 300 μL lysis buffer and kept on ice for 20 min and lysates were cleared by centrifugation. Approximately 5% of the cleared lysates was used for input and the remaining lysate was added to 20 μl of washed Glutathione Sepharose 4 Fast flow beads (GE Healthcare) for capture of GST-TUBE2 and bound material. Reactions were kept at 4 °C with rotation for 1–2 h, followed by 4 × washing in 500 μl of ice-cold TBS containing 0.1% Tween20 (TBS-T). Bound material was separated from beads by addition of 1 × LSB and analyzed on SDS–PAGE for the indicated proteins. PCR assay PCR was used to detect the expression of Nox gene expression in SKOV3 cells. RNA was purified according to standard protocol (Qiagen) and reverse transcribed into complementary DNA (cDNA; Qiagen). PCR was performed in 50 μl of 10 mmol l −1 Tris-HCl (pH 8.3), 25 mmol l −1 MgCl 2 , 10 mmol l −1 dNTP, 100 U of Taq DNA polymerase, with 0.1 μmol l −1 each primer and was terminated by heating at 70 °C for 15 min. PCR products were resolved on a 1% agarose gel and visualized with ultraviolet light after ethidium bromide treatment. The following primers ware used (5′–3′): human Nox1 sense, CTTCCTCACCGGATGGGACA; human Nox1 antisense, TGACAGCATTTGCGCAGGCT; human Nox2 sense, CCTGTACCTGGCTGTGACCCTGTT; human Nox2 antisense, ACCCCAATCCCTGCTCCCACTAA; human Nox3 sense, GAGTGGCACCCCTTCACCCT; human Nox3 antisense, CTAGAAGCTCTCCTTGTTGT; human Nox4 sense, AGTCAAACAGATGGGATA; human Nox4 antisense, TGTCCCATATGAGTTGTT; human Nox5 sense, AAGCATACTTGCCCCAGCTG; human Nox5 antisense, CAGGCCAATGGCCTTCATGT. Microscopy All microscopy was performed on a HAL100 Zeiss microscope. Image acquisition and analysis was carried out with LSM-ZEN software and ImageJ. Zebrafish Hace1 model Zebrafish were maintained, bred and developmentally staged as described [58] . The Dalhousie University Animal Care Committee approved use of zebrafish in this study. The hace1 - HECT morpholino (5′-CCCTCGAACTGTTAGACAGAATAAA)-3′ and standard control morpholino (5′-CCTCTTACCTCAGTTACAATTTATA)-3′ were purchased from Genetools LLC (Philomath, OR). The hace1 - HECT morpholino targets a splice site which resides within the catalytically active HECT domain, and is positioned upstream of the critical cysteine residue (C876S) required for hace1 ubiquitin ligase function. Morpholinos were diluted to a working concentration of 1.6 mM with 1% phenol red, and were injected into live zebrafish embryos at the 1–4 cell stage. Digoxigenin- and fluorescein isothiocyanate (FITC)-labeled antisense RNA probes were transcribed from linearized cDNA constructs according to the manufacturer’s protocols (Roche Molecular Biochemicals, Indianapolis, IN). Whole-mount in situ hybridization assays for zebrafish embryos were conducted as described [59] . Staining was performed using BCIP/NBT (Vector laboratories, Burlington, ON, Canada). The Hace1 morpholino was verified by reverse transcription–PCR using the following primers (5′–3′): Primer A: forward 5′-TTGCTGGTCAAATCCTGGGTCTGG-3′; Reverse-5′-AATGCAGTGCGACAAGCAAGCG-3′; Primer B: Forward-5′-AGCCAGGAGGAACTACCATTCAGG-3′; Reverse-5′-ATAACTCCCACAATGCAGTGCGAC-3′. Single Whole-mount in situ hybridization images were taken on a Leica MZ16F with a DFC 490 camera. Double fluorescence in situ experiments were performed with Fast Red (Vector laboratories) staining, and then imaged with a Zeiss Observer Z.1 microscope with a Colibri fluorescence source. H 2 O 2 imaging using a live cell fluorescein dye was adapted from a previously described assay [60] . In brief, 48 h post fertilization (hpf) casper embryos were loaded for 30 min with 50 μM pentafluorobenzenesulphonyl fluorescein (Cayman Chemical) in 1% dimethylsulphoxide in egg water, and imaged using a 550-nm bandpass filter. Where indicated, the morpholinos were incubated for 1 h with 100 μM DPI or 24 h with 200 μM APO. Zebrafish embryos were dissociated to a single-cell suspension, and sorted on a FACSAria I (BD Biosciences, San Jose, CA, USA). Cells were thresholded by forward scatter (FSC) and side scatter (SSC) and interrogated by Coherent Sapphire solid state 488 nm laser with dual bandpass filter including FITC (515–545 nm) emission. ROS + cells were gated by the following parameters: FSC LO and SSC LO , and FITC HI fluorescence. Statistical tests When indicated, data were subjected a two-tailed Student’s t -test to resolve statistical significance. Data compiled from several experiments are presented with a ±s.e.m. Human and murine tissue material Snap-frozen matched tissue specimens of human normal kidney and Wilms’ tumor from the same patients were obtained from the Children’s Oncology Group Wilms’ tumor tissue bank, kindly contributed by Dr Paul Grundy, Cross Cancer Centre, Edmonton, Alberta. Snap-frozen murine tumors were obtained from wild-type and Hace1 knockout mice at the BC Cancer Research Centre. The British Columbia Cancer Agency and UBC ethical committees have approved the use of human tissue specimens and mouse models in this study. All specimens were cut in 20 μm sections at −20 °C using a cryostat, mounted on cover slides on dry ice, washed in ice-cold HBSS, and immediately DHE-treated as described for cell lines and analyzed for oxyethidium light emission by microscopy. In parallel, 5 μm sections were cut and haematoxylin and eosin stained for verification of tissue integrity and pathology. All tumor sections contained at least 80% viable tumor tissue. In cases with sufficient tissue available, additional sections were cut for preparing protein lysates to be analyzed by SDS–PAGE for the indicated proteins. Wilms’ tumors used in this study were chosen on the basis of having been previously shown to have low or undetectable Hace1 mRNA and protein expression as measured by reverse transcription–PCR or western blotting, respectively [6] . How to cite this article: Daugaard, M. et al . Hace1 controls ROS generation of vertebrate Rac1-dependent NADPH oxidase complexes. Nat. Commun. 4:2180 doi: 10.1038/ncomms3180 (2013)